Griffiths phases and the stretching of criticality in brain networks Hallmarks of criticality, such as power-laws and scale invariance, have been empirically found in cortical-network dynamics and it has been conjectured that operating at criticality entails functional advantages, such as optimal computational capabilities, memory and large dynamical ranges. As critical behaviour requires a high degree of fine tuning to emerge, some type of self-tuning mechanism needs to be invoked. Here we show that, taking into account the complex hierarchical-modular architecture of cortical networks, the singular critical point is replaced by an extended critical-like region that corresponds—in the jargon of statistical mechanics—to a Griffiths phase. Using computational and analytical approaches, we find Griffiths phases in synthetic hierarchical networks and also in empirical brain networks such as the human connectome and that of Caenorhabditis elegans . Stretched critical regions, stemming from structural disorder, yield enhanced functionality in a generic way, facilitating the task of self-organizing, adaptive and evolutionary mechanisms selecting for criticality. Empirical evidence that living systems can operate near critical points is flowering in contexts ranging from gene expression patterns [1] , to optimal cell growth [2] , bacterial clustering [3] or flocks of birds [4] . In the context of neuroscience, synchronization patterns have been shown to exhibit broadband criticality [5] , critical avalanches of spontaneous neural activity have been consistently found both in vitro [6] , [7] , [8] and in vivo [9] , and results from large-scale brain models based on the human connectome show that only at criticality the brain structure is able to support the dynamics observed in functional magnetic resonance imaging (fMRI) recordings [10] . All this evidence suggests that criticality—with its concomitant power-laws and scale invariance–might have a relevant role in intact–brain dynamics [8] , [11] . At variance with inanimate matter—for which the emergence of generic or self-organized criticality in sandpile models, type-II superconductors or solar flares is relatively well understood [12] , [13] , [14] —criticality in living systems can be conjectured to be the result of evolutionary or adaptive processes, which for reasons to be understood select for it. The criticality hypothesis [8] , [11] , [15] states that biological systems can perform the complex computations that they require to survive only by operating at criticality (the edge-of-chaos), that is, at the borderline between an active or chaotic phase in which noise propagates unboundedly—thereby corrupting all information processing or storage—and a quiescent or ordered phase in which perturbations readily fade away, hindering the ability to react and adapt [16] , [17] . Critical dynamics provides a delicate trade-off between these two impractical tendencies, and it has been argued to imply optimal transmission and storage of information [7] , [8] , [18] , optimal computational capabilities [19] , large network stability [17] , maximal variety of memory repertoires [20] and maximal sensitivity to stimuli [21] . Such a delicate balance occurs just at a singular or critical point, requiring a precise fine tuning. However, a very recent fMRI analysis of the human brain at its resting state reveals that the brain spends most of the time wandering around a broad region near a critical point, rather than just sitting at it [22] . This suggests that the region where cortical networks operate is not just a critical point, but a whole extended region around it. Here inspired by this empirical observation as well as by some recent findings in network theory and neuroscience [23] , [24] , [25] , we scrutinize the dynamics of simple models of neural activity propagation when the structural architecture of brain networks is explicitly taken into account. Using a combination of analytical and computational tools, we show that the intrinsically disordered (hierarchical and modular) organization of brain networks dramatically influences the dynamics by inducing the emergence—in the jargon of Statistical Mechanics—of a Griffiths phase (GP) [23] , [26] , [27] , [28] . This phase, which stems from the presence of disorder (structural heterogeneity here), is characterized by generic power-laws extending over broad regions in parameter space. Furthermore, functional advantages usually ascribed to criticality, such as a huge sensitivity to stimuli, are reported to emerge generically all along the GP. Remarkably, not only do we find GPs in stylized models of brain architecture, but also in real neural networks such as those of the Caenorhabditis elegans ( C. elegans ) and the human connectome. Our conclusion is that, as a consequence of the intrinsically disordered architecture of brain networks, critical-like regions are extended from a singular point to a broad or stretched region, much as evidenced in recent fMRI experiments. The existence of GPs facilitates the task of self-organizing, adaptive or evolutive mechanisms seeking for critical-like attributes, with all their alleged functional advantages. We claim that the intrinsic structural heterogeneity of cortical networks calls for a change of paradigm from the critical/edge-of-chaos to a new one, relying on extended critical-like Griffiths regions. Our work also raises a series of questions worthy of future pursuit. For instance, is there any connection between GPs and the empirically reported generic power-law decay of short-time memories? Do our results extend to other hierarchical architectures such as those encountered in metabolic or technological networks? Hierarchical network architectures The cortex network has been the focus of attention in neuroanatomy for a long time, but only recently the development of high-throughput methods has allowed the unveiling of its intricate architecture or connectome [29] , [30] . Brain networks have been found to be structured in moduli—each modulus being characterized by having a much denser connectivity within it than with elements in other moduli—organized in a hierarchical fashion across many scales [31] , [32] , [33] . Moduli exist at each hierarchical level: cortical columns arise at the lowest level, cortical areas at intermediate ones and brain regions emerge at the systems level, forming a sort of fractal-like nested structure [31] , [32] , [33] , [34] . To be able to perform systematic analyses, we have designed synthetic hierarchical and modular networks (HMN) with s hierarchical levels, N nodes/neurons and L links/synapses, whose structure can be tuned to mimic that of real networks. We employ two different HMN models based on a bottom–top approach; in the first, local fully connected moduli are constructed and then recursively grouped by establishing new inter-moduli links between them in either a stochastic way with a level-dependent probability p as sketched in Fig. 1 (HMN-1) section or in a deterministic way with a level-dependent number of connections (HMN-2). For further details see the Methods section. Similarly, top–down models can also be designed [35] . 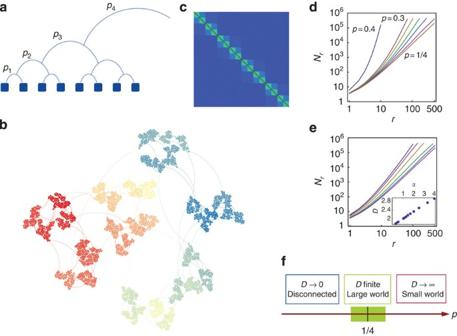Figure 1: Hierarchical-modular networks. (a) Sketch of the bottom–top approach (HMN-1 model): initially, nodes are grouped into fully connected modules of sizeM0(blue squares); then nodes in different modules are clustered recursively into sets ofbhigher level blocks (for example, in pairs,b=2) linking their respective nodes with hierarchical level-dependent wiring probabilities (HMN-1):pl=αplwith 0<p<1 and α a constant. At levell, each of the existingN/2lpairs is connected on average bynl=4l(M0/2)2× αpllinks. The resulting networks are always connected; with total number ofN=M0×bsnodes, and average connectivity. (b) Graph representation of a HMN-1 withN=211nodes, organized acrosss=10 hierarchical levels (M0=2,p=1/4, andα=4). (c) Adjacency matrix of the connection-density (as inb) averaged over several network realizations (greener for larger densities). (d,e) Topological dimension,D, as defined byNr~rD(see main text) as a function of parameters. (d) Aspis increasedD(the slope of the straight lines in the double logarithmic plot) grows and eventually becomes infinite; for smaller values ofp(not shown) it becomes flat, andD→0. (e) Keepingp=1/4, the topological dimensionDis finite and continuously varying as function ofα, (values summarized in the inset). (f) Summary of structural properties: networks are disconnected (vanishing topological dimension,D) and small-world (D=∞) for small and large values ofp, respectively, while aroundp=1/4 networks have a finiteD(as well as a finite connectivity and a finite density of connections in the large-Nlimit, that is, networks are scalable). Figure 1: Hierarchical-modular networks. ( a ) Sketch of the bottom–top approach (HMN-1 model): initially, nodes are grouped into fully connected modules of size M 0 (blue squares); then nodes in different modules are clustered recursively into sets of b higher level blocks (for example, in pairs, b =2) linking their respective nodes with hierarchical level-dependent wiring probabilities (HMN-1): p l =α p l with 0< p <1 and α a constant. At level l , each of the existing N /2 l pairs is connected on average by n l =4 l ( M 0 /2) 2 × α p l links. The resulting networks are always connected; with total number of N = M 0 × b s nodes, and average connectivity . ( b ) Graph representation of a HMN-1 with N =2 11 nodes, organized across s =10 hierarchical levels ( M 0 =2, p =1/4, and α =4). ( c ) Adjacency matrix of the connection-density (as in b ) averaged over several network realizations (greener for larger densities). ( d , e ) Topological dimension, D , as defined by N r ~ r D (see main text) as a function of parameters. ( d ) As p is increased D (the slope of the straight lines in the double logarithmic plot) grows and eventually becomes infinite; for smaller values of p (not shown) it becomes flat, and D →0. ( e ) Keeping p =1/4, the topological dimension D is finite and continuously varying as function of α , (values summarized in the inset). ( f ) Summary of structural properties: networks are disconnected (vanishing topological dimension, D ) and small-world ( D =∞) for small and large values of p , respectively, while around p =1/4 networks have a finite D (as well as a finite connectivity and a finite density of connections in the large- N limit, that is, networks are scalable). Full size image A way to encode key network structural information is the topological dimension, D , that measures how the number of neighbours of any given node grows when moving 1, 2, 3,..., r steps away from it: N r ~ r D for large values of r . Networks with the small-world property [36] have local neighbourhoods quickly covering the whole network, that is, N r grows exponentially with r , formally corresponding to D →∞. Instead, large-worlds have a finite topological dimension, while D =0 describes fragmented networks (see Fig. 1 ). Our synthetic HMN models span all the spectrum of D -values as illustrated in Fig. 1 . Strictly speaking, the HMN networks that we will consider in the following are finite dimensional only for p =1/4, in which case the number of inter-moduli connection is stable across hierarchical levels (see Methods). For p> 1/4 (resp. p< 1/4), networks become more and more densely (resp. sparsely) connected as the hierarchy depth (that is, the network size) is increased. Deviations from p =1/4 create fractal-like networks up to certain scale, being good approximations for finite-dimensional networks in finite size. In some works (for example, Gallos et al. [37] ), the Hausdorff (fractal) dimension D f is computed for complex networks. We have verified numerically that D f ≈ D in all cases for HMNs. Architecture-induced GPs Disorder is well-known to radically affect the behaviour of phase transitions (see studies by Vojta [28] and references therein). In disordered systems, there exist local regions characterized by parameter values that differ significantly from their corresponding system averages. Such rare-regions can, for instance, induce the system to be locally ordered, even if globally it is in the disordered phase. In this way, in propagation-dynamic models, activity can transitorily linger for long times within rare active regions, even if the system is in its quiescent phase. In the particular case in which broadly different rare-regions exist—with broadly distinct sizes and time-scales—the overall system behaviour, determined by the convolution of their corresponding highly heterogeneous contributions, becomes anomalously slow (see below). In contrast with standard critical points, systems with rare-region effects have an intermediate broad phase separating order from disorder: a GP with generic power-law behaviour and other anomalous properties (see studies by Vojta [28] and below). Remarkably, it has been very recently shown that structural heterogeneity can have, in networked systems, a role analogous to that of standard quenched disorder in physical systems [23] . In particular, simple dynamical models of activity propagation exhibit GPs when running upon networks with a finite topological dimension D . On the other hand, in small-world networks (with D =∞) local neighbourhoods are too large—quickly covering the whole network—as to be compatible with the very concept of rare (isolated) regions [23] . Therefore, it has been conjectured that a finite topological dimension D is an excellent indicator of eventual rare-region effects and GPs. Anomalous propagation dynamics in HMNs To model the propagation of neuronal activity, we consider highly simplified dynamical models running upon HMNs. More realistic models of neural dynamics with additional relevant layers of information could be considered, but we do not expect them to significantly affect our conclusions. Our approach here consists in modelling activity propagation in a minimal way; in some of the cases that we study, the network nodes are not neurons but coarse neural regions, for which effective models of activity propagation are expected to provide a sound description of large-scale properties. Every node (or neuron) is endowed with a binary state variable σ , representing either activity ( σ =1) or quiescence ( σ =0). Each active neuron is spontaneously deactivated at some rate μ ( μ =1 here), while it propagates its activity to other directly connected neurons at rate λ. We have considered two different dynamics: in the first one, (Model A) a synapsis between an active and a quiescent node is randomly selected at each time and proved for activation, while in the other variant (Model B) a neuron is selected and all its neighbours are proved for activation. Details of the computational implementation of the two models, known in statistical physics as the contact process and the SIS model respectively, can be found in Methods. In general, depending on the value of λ , these models can be either in an active phase—for which the density ρ of active nodes reaches a steady-state value ρ s >0 in the large system size and large-time limit—or in the inactive phase in which ρ falls ineluctably in the quiescent configuration ( ρ s =0). Separating these two regimes, at some value, λ c , there is a standard critical point where the system exhibits power-law behaviour for quantities of interest, such as the time decay of a homogeneous initial activity density, ρ ( t )~ t − θ , or the size distribution of avalanches triggered by an initially localized perturbation, P ( S )~ S − τ . Here θ and τ are critical indices or exponents. This standard critical-point scenario (see Fig. 2a,b ) holds for regular lattices, Erdös-Renyi networks and many other types of networks. On the other hand, computer simulations of the different dynamical models running upon our complex HMN topologies with finite D reveal a radically different behaviour (see Fig. 2c–f and Methods). The power-law decay of the average density ρ ( t )—specific to the critical point in pure systems—extends to a broad range of λ values. The existence of a broad interval with power-law decaying activity is supported by finite size scaling analyses reported in Methods. Likewise, as shown in Fig. 2f , avalanches of activity generated from a localized seed have power-law distributed sizes, with continuously varying exponents, in the same broad region. These features are fingerprints of a GP and have been confirmed to be robust against increasing system size (up to N =2 20 ), using different types of HMN (HMN-1 with different values of α and p , HMN-2 models, all with finite D ) and dynamical models (see Methods). 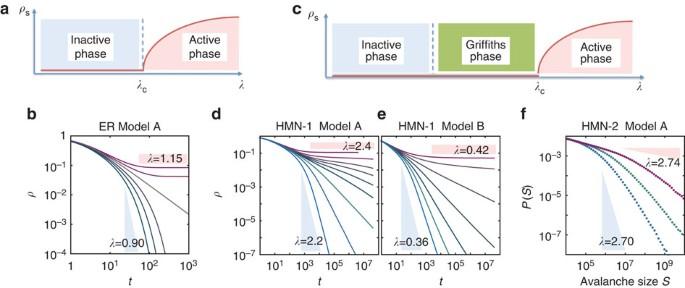Figure 2: Conventional versus non-conventional phase diagram. Left: (a,b) Conventional critical point scenario for our Model A running upon a random Erdös–Rényi network (106nodes, average connectivity 20, infinite topological dimensionD): a singular power-law separates a quiescent phase (with exponential decay) from an active one (with a non-trivial steady-state). Right: (c–f) Emergence of broad regions of power-law scaling in HMNs. (c) Schematic phase diagram for a system exhibiting a broad region of power-law scaling. The stationary density of activity,ρs, is depicted as a function of the spreading rate λ. (d,e) Steady-state density of active sites for Model A and Model B dynamics, respectively, on HMN-1 networks (withN=214nodes, and parameterss=13,p=1/4,α=1). Data for increasing values of the spreading rateλ, from bottom to top. (f) Avalanche-size distributions for Model A on a HMN-2 network (N=214,s=13,p=1/4,α=1; GP for such networks is observed for 2.60≤λ≤2.79); avalanche sizes are power-law distributed over a wide-rangeλvalues reflecting the existence of a GP. These conclusions have been confirmed in finite-size scaling analyses, and can be generalized for other combinations of network architectures and dynamical models. Figure 2: Conventional versus non-conventional phase diagram. Left: ( a , b ) Conventional critical point scenario for our Model A running upon a random Erdös–Rényi network (10 6 nodes, average connectivity 20, infinite topological dimension D ): a singular power-law separates a quiescent phase (with exponential decay) from an active one (with a non-trivial steady-state). Right: ( c – f ) Emergence of broad regions of power-law scaling in HMNs. ( c ) Schematic phase diagram for a system exhibiting a broad region of power-law scaling. The stationary density of activity, ρ s , is depicted as a function of the spreading rate λ. ( d , e ) Steady-state density of active sites for Model A and Model B dynamics, respectively, on HMN-1 networks (with N =2 14 nodes, and parameters s =13, p =1/4, α =1). Data for increasing values of the spreading rate λ , from bottom to top. ( f ) Avalanche-size distributions for Model A on a HMN-2 network ( N =2 14 , s =13, p =1/4, α =1; GP for such networks is observed for 2.60≤ λ ≤2.79); avalanche sizes are power-law distributed over a wide-range λ values reflecting the existence of a GP. These conclusions have been confirmed in finite-size scaling analyses, and can be generalized for other combinations of network architectures and dynamical models. Full size image How do Griffith phases work? For illustration purposes, let us consider a simplified example. Consider Model A (the contact process) on a generic network, with a node-dependent quenched spreading rate λ ( x ), characterized—without loss of generality—by a bimodal distribution of λ with average value . Suppose, the two possible values of λ are one above and one below the critical point of the pure model, λ c . In this way, at each location the system has an intrinsic preference to be either in the active or in the quiescent phase. Under these circumstances, typically, λ c < c , so that, for values of in between λ c and c the disordered system is in its quiescent phase. However, there are always spatial locations characterized by significantly over-average values of (actually, local values of λ ( x )> λ c ). In these regions, initial activity can linger for very long periods, especially if they happen to be large. Still, as such rare-regions have a finite size, they ineluctably end up falling into the inactive state. Considering a rare active region of size ζ , it decays to the quiescent state after a typical time τ ( ζ ), which grows exponentially with cluster size, that is, τ ≃ t 0 exp[ A (λ)ζ] (Arrhenius law), where t 0 and A (λ) do not depend on ζ . On the other hand, the distribution of ζ -values is also exponential (very large regions are exponentially rare). Therefore, the overall activity density, ρ ( t ), decays as the following convolution integral which evaluated in saddle-point approximation leads to ρ ( t )~ t − θ , with θ ( ) varying continuously with the disorder average value, . Such generic power-laws signal the emergence of GPs. This is just an explanatory example of a general phenomenon, thoroughly studied in classical, quantum and non-equilibrium disordered systems [28] . In HMNs, the quenched disorder is encoded in the intrinsic disorder of the hierarchical contact pattern. Diverging response in HMNs One of the main alleged advantages of operating at criticality is the strong enhancement of the system’s ability to distinctly react to highly diverse stimuli. In the statistical mechanics jargon, this stems from the divergence of the susceptibility at criticality [38] . How do systems with broad GPs respond to stimuli? To answer this question we measure the following two different quantities (see Methods): First, the dynamic susceptibility gauges the overall response to a continuous localized stimulus and is defined as Σ( λ )= N [ ρ f ( λ )– ρ s ( λ )], where ρ s ( λ ) is the stationary density in the absence of stimuli and ρ f ( λ ) is the steady-state density reached when one single node is constrained to remain active. As shown in Fig. 3 , Σ becomes extremely large in the GP and, more importantly, it grows as a power-law of system size, Σ( λ ≈ λ c , N )~ N η , implying that there is an extended extended region (the whole GP) where the system exhibits a divergent response (with λ -dependent continuously varying exponents). 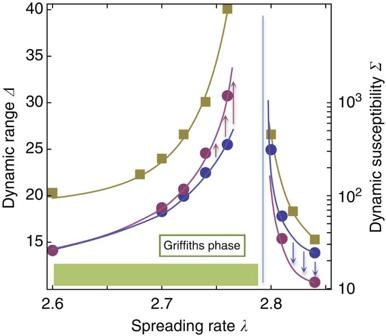Figure 3: Network response diverges all along the GP. Right axis: dynamic susceptibility,Σ, measured for the dynamical Model A in HMN-2 networks of sizeN=214(blue circles) andN=217(purple circles); the critical pointλc≈2.79 is marked as a vertical line (see Methods: dynamical protocol iii). In the GP (resp. active phase), the overall response increases (resp. decreases) for larger systems as marked by the red (resp. blue) arrows. In the GP,Σgrows as a λ-dependent power-law ofN. Left axes: dynamic range Δ (green squares) for the same case as above,N=214(dynamical protocol iv; see Methods). Instead of the usual symmetric cusp-singularity at the critical point, there is a whole region of extremely large Δ with a strong asymmetry around the transition point, as corresponds to the existence of a GP. Figure 3: Network response diverges all along the GP. Right axis: dynamic susceptibility, Σ , measured for the dynamical Model A in HMN-2 networks of size N =2 14 (blue circles) and N =2 17 (purple circles); the critical point λ c ≈2.79 is marked as a vertical line (see Methods: dynamical protocol iii). In the GP (resp. active phase), the overall response increases (resp. decreases) for larger systems as marked by the red (resp. blue) arrows. In the GP, Σ grows as a λ-dependent power-law of N . Left axes: dynamic range Δ (green squares) for the same case as above, N =2 14 (dynamical protocol iv; see Methods). Instead of the usual symmetric cusp-singularity at the critical point, there is a whole region of extremely large Δ with a strong asymmetry around the transition point, as corresponds to the existence of a GP. Full size image Second, the dynamic range, Δ, introduced in this context in the studies by Kinouchi and Copelli [21] measures the range of perturbation intensities/frequencies for which the system reacts in distinct ways, being thus able to discriminate among them. We have computed Δ( λ ) in the HMN-2 model (see Fig. 3 ), which clearly illustrates the presence of a broad region with huge dynamic ranges (rather than the standard situation for which large responses are sharply peaked at criticality). Therefore, if critical-like dynamics is important to access a broad dynamic range and to enhance system’s sensitivity, then it becomes much more convenient to operate with hierarchical-modular systems, where criticality—with extremely large responses and huge sensitivity—becomes a region rather than a singular point. GPs in real networks Analyses of different nature have revealed that organisms from the primitive C. elegans [32] , [33] , [39] , [40] (for which a full detailed map of its about 300 neurons has been constructed) to cats, macaque monkeys or humans (for which large-scale connectivity maps are known [29] ) have a hierarchically organized neural network. Such structure is also shared by functional brain networks (for example, from fMRI data) [29] , [30] , [37] , [41] , [42] . Do simple dynamical models of activity propagation (such as those in previous sections) running upon real neural networks exhibit GPs? We have considered the human connectome network, obtained by Sporns and collaborators [29] , [30] using diffusion imaging techniques. It consists of a highly coarse-grained mapping (as opposed for instance to the detailed map of C. elegans ) of anatomical connections in the human brain, comprising N =998 brain areas and the fibre tract densities between them, with a hierarchical organization [32] , [33] (see Methods). Given that this network comprises only N ≲ 1,000 nodes, the maximum size of possible rare-regions and the associated power-laws are necessarily cutoff at small sizes and short times. Nevertheless, as illustrated in Fig. 4 , simulations of the dynamical models above (Model B in this case) show a significant deviation from the typical standard critical-point scenario. Instead, avalanches are clearly distributed as power-laws, with moderate finite-size effects, in a broad range of λ -values (see Fig. 4 ). Actually, truncated power-laws of the form P ( S )~ S − τ e −S/ξ —with λ-dependent values of τ —provide highly reliable fits of the size distributions, P ( S ), according to the Kolmogorov–Smirnoff criterion (see Methods), supporting the picture of a broad critical-like region. This strongly suggests that if it were feasible to run dynamical models upon the actual human brain network (with about 10 12 neurons and 10 15 synapses) a GP would appear in a robust way, and would extend over much larger range of size and time scales. Similar results, even if affected by more severe size effects, are obtained for the C. elegans detailed neural network consisting of N ≲ 300 neurons (see Fig. 4 , upper inset). 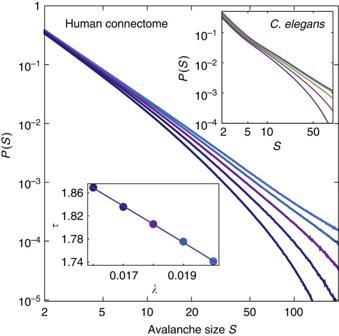Figure 4: Critical avalanches all along the GP in real brain networks. Avalanche-size statistics for Model B dynamics in real neural networks. Main plot: human connectome network (consisting of 998 brain areas and the structural connections among them). Avalanche-size distributions for Model B dynamics (with 0.016≤λ≤0.020 equispaced values). Truncated power-lawsP(S)~S−τe−S/ξwith continuously varying exponentsτconstitute the most reliable fits according to the Kolmogorov–Smirnoff criterion (see Methods). Lower inset: Theτexponent (estimated through non-linear least-square fits) as a function of λ; it converges to ≈1.7 at the critical point,λc≈0.020. Upper inset: as the main figure but for theC. elegansneural network (0.08≤λ≤0.12). Figure 4: Critical avalanches all along the GP in real brain networks. Avalanche-size statistics for Model B dynamics in real neural networks. Main plot: human connectome network (consisting of 998 brain areas and the structural connections among them). Avalanche-size distributions for Model B dynamics (with 0.016≤ λ ≤0.020 equispaced values). Truncated power-laws P ( S )~ S −τ e − S /ξ with continuously varying exponents τ constitute the most reliable fits according to the Kolmogorov–Smirnoff criterion (see Methods). Lower inset: The τ exponent (estimated through non-linear least-square fits) as a function of λ; it converges to ≈1.7 at the critical point, λ c ≈0.020. Upper inset: as the main figure but for the C. elegans neural network (0.08≤ λ ≤0.12). Full size image Spectral fingerprints of GPs in HMNs To further confirm the existence of GPs (beyond direct computational simulations), here we present some analytical results. An important tool in the analysis of network dynamics is provided by spectral graph theory, in which the network structure is encoded in some matrix and linear algebra techniques are exploited [43] . For instance, the dynamics of simple models (for example, Model B) is often governed by the largest (or principal) eigenvalue, Λ max , of the adjacency matrix, A ij (with 1’s as entries for existing connections and 0’s elsewhere), which straightforwardly appears in a standard linear stability analysis (as detailed in the Methods section). It is easy to show that (with very mild assumptions) the critical point—signalling the limit of linear stability of perturbations on the quiescent state—is given by λ c Λ max =1. Remarkably, it has been recently shown that this general result may not hold for certain networks, for which the largest eigenvalue has an associated localized eigenvector (for example, with only a few non-vanishing components; this phenomenon closely resembles Anderson localization in physics [44] ). In such a case, linear instabilities for λ slightly larger than 1/Λ max lead to localized activity around only few nodes (where the corresponding eigenvector is localized), not pervading the network and not leading to a true active state. This implies that the critical point is shifted to a larger value of λ . Instead, these regions of localized activity resemble very much rare-regions in GPs: activity lingers around them until eventually a large fluctuation kills them. Inspired by this novel idea, we performed a spectral analysis of our HMNs (for example, HMN-2 nets with α =1, see Fig. 5 ), with the result that—for finite D networks—not only the largest eigenvalue Λ max corresponds to a localized eigenvector, but a whole range of eigenvalues below Λ max (even hundreds of them) share this feature, as can be quantitatively confirmed (see Fig. 5c, d and Methods). In particular, the principal eigenvector is heavily peaked around a cluster of neighbouring nodes. We have conjectured and verified numerically that the clusters where the largest eigenvalues are localized correspond to the rare-regions, with above-average connectivity and where localized activity lingers for long time. Also, we numerically found λ c ≈0.41>1/ Λ max ≈0.33 confirming the prediction above. The interval between these two values defines the GP (see Methods). 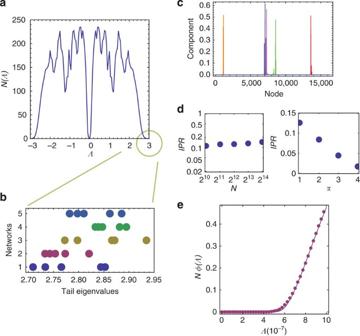Figure 5: Spectral analyses of hierarchical networks. (a) Average spectrum of the adjacency matrix of HMN-2 networks (N=214,s=13,M0=2,α=1). Data are averaged over 150 network realizations. The vertical axis reports the average number of eigenvalues (not the density). (b) Ideal zoom of the higher spectral edge of (a). The values of the five largest eigenvalues for five randomly chosen networks from (a) are represented. No proper spectral gap is observed. (c) Localization of the five eigenvectors corresponding to the largest eigenvalues. The principal eigenvectorf(Λmax) is plotted in red. Being our HMNs connected, in agreement with the Perron–Frobenius theorem60, the components off(Λmax) (even the vanishing ones) are all strictly positive, although this cannot be appreciated in linear scale. The next eigenvectors are plotted in magenta, orange, green and blue. (d) Dependence of the IPR on the system size and the number of block-block connections in HMN-2 networks. (e) Lower spectral edge of the cumulative distribution of Laplacian eigenvalues of HMN-2 networks as in (a). Numerical data (points) are compared with an exponential Lifshitz tail with exponenta≈1.00. The Laplacian matrix is defined as. Figure 5: Spectral analyses of hierarchical networks. ( a ) Average spectrum of the adjacency matrix of HMN-2 networks ( N =2 14 , s =13, M 0 =2, α =1). Data are averaged over 150 network realizations. The vertical axis reports the average number of eigenvalues (not the density). ( b ) Ideal zoom of the higher spectral edge of ( a ). The values of the five largest eigenvalues for five randomly chosen networks from ( a ) are represented. No proper spectral gap is observed. ( c ) Localization of the five eigenvectors corresponding to the largest eigenvalues. The principal eigenvector f ( Λ max ) is plotted in red. Being our HMNs connected, in agreement with the Perron–Frobenius theorem [60] , the components of f ( Λ max ) (even the vanishing ones) are all strictly positive, although this cannot be appreciated in linear scale. The next eigenvectors are plotted in magenta, orange, green and blue. ( d ) Dependence of the IPR on the system size and the number of block-block connections in HMN-2 networks. ( e ) Lower spectral edge of the cumulative distribution of Laplacian eigenvalues of HMN-2 networks as in ( a ). Numerical data (points) are compared with an exponential Lifshitz tail with exponent a ≈1.00. The Laplacian matrix is defined as . Full size image In addition, we also considered large network ensembles and computed the probability distribution of eigenvalues. We found that the distribution of the eigenvalues corresponding to localized eigenvectors results in an exponential tail of the continuum spectrum, where an infinite dimensional graph would exhibit a spectral gap instead (see Methods). This translates into an exponential tail of the cumulative distribution φ ( Λ ) of Laplacian eigenvalues (or integrated density of states) at the lower spectral edge, a so-called Lifshitz tail—which in equilibrium systems is related to the Griffiths singularity [45] . We have found Lifshitz tails with their characteristic form (where a is a real parameter, see Fig. 5e ). Interestingly, Lifshitz tails are also rigorously predicted on Erdös Rényi networks below the percolation threshold, where rare-region effects and GPs are an obvious consequence of the network disconnectedness [46] . Therefore, the presence of both (i) localized eigenvectors and (ii) Lifshitz tails confirms the existence of GPs in networks with complex heterogeneous architectures. The fingerprints of extended criticality in the human connectome are a result of its hierarchical network structure, and the localization properties that characterize it. 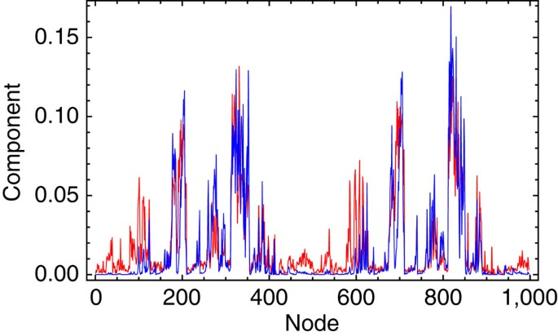Figure 6: Localization properties of the human connectome network. Principal eigenvector of the weighted (blue) and unweighted (red) adjacency matrix. As the peak structure is roughly preserved, localization properties are expected to be alike in the two representations. In both cases regions of localized activity are evident. Figure 6 supports this view highlighting the localization of the principal eigenvector. In particular, we show that the principal eigenvector of the full adjacency matrix and that of the unweighted (that is, with 1’s as entries in correspondence to every non-zero weight) version of it display very similar peak structures (that is, their rare-regions are very similar). This last observation supports our choice to run simple unweighted dynamics on top of the connectome network. Connection weights will certainly contribute to a fully realistic description of the brain function, but they are not necessary in order to achieve broad criticality, which primarily arises from structural disorder. Figure 6: Localization properties of the human connectome network. Principal eigenvector of the weighted (blue) and unweighted (red) adjacency matrix. As the peak structure is roughly preserved, localization properties are expected to be alike in the two representations. In both cases regions of localized activity are evident. Full size image A few pioneering studies have recently explored the role of hierarchical-modular networks (HMN) on different aspects of neural dynamics. Rubinov et al. [24] argued that HMNs have a crucial role in fostering the existence of critical dynamics. Similar observations have been also made for spreading dynamics [35] , [47] , [48] and for self-organization models [25] , but so far these remain empirical findings lacking a satisfactory explanation. Aimed at shedding light on these issues, here we have made the conjecture that owing to the intrinsically heterogeneous (that is, disordered) architecture of brain HMNs and their large-world nature (which implies finite topological dimensions D ), GPs are expected to emerge. These are characterized by broad regions in parameter space exhibiting critical-like features and, thus, not requiring of a too-precise fine tuning. To confirm this claim, we use a combination of computational tools and analytical arguments. In particular, we have constructed different synthetic HMNs covering a broad range of architectures (with either large- or small-world properties). For large-worlds (that is, finite topological dimension D ), we find ( i ) generic anomalous slow relaxation and power-law distributed avalanches (with continuously varying exponents) in a broad region comprised between the active and the inactive phase; ( ii ) the system’s response to stimuli (as measured by the dynamic susceptibility and the dynamic range) is anomalously large: it diverges with system size through the whole GP. At a theoretical level, graph-spectral analyses reveal the presence of localized eigenvectors and Lifshitz tails, which are the spectral counterparts of rare-regions and GPs. All these evidences confirm the existence of GPs in synthetic HMNs, including a spectral graph theory viewpoint, thereby going beyond previous results in generic complex networks [23] . More remarkably, we have also provided evidence that GPs appear in actual real networks such as those of the human connectome and C. elegans , even if owing to the limited available network-sizes the associated power-laws are necessarily cutoff. Still, the best fits to data are provided by continuously varying power-laws, truncated by finite-size effects. It is noteworthy that disorder needs to be present at very different scales for GPs to emerge (otherwise rare-regions cannot be arbitrarily large); this is why a hierarchy of levels is required. Plain modular networks—without the broad distribution of cluster sizes, characteristic of hierarchical structures—are not able to support GPs. We emphasize that GPs in HMNs are induced merely by the existence of structural disorder: no additional form of neuronal or synaptic heterogeneity has been considered here; adding further heterogeneity would only enhance rare-region effects and hence GPs. For instance, we have also found GPs for the human connectome, when taking into account the relative weight of structural connections. It should also be noticed that all networks in our study are undirected in the sense that links are symmetrical, although synapses in cortical networks are not. Again, this does not jeopardize our conclusions: directness in the connections only strengthens isolation and hence rare-region effects and GPs. The existence of a GP with its concomitant generic power-law scaling—not requiring a delicate parameter fine tuning—provides a more robust and solid basis to justify the ubiquitous presence of scale-free behaviour in neural data, from EEG or MEG records to neural avalanches. More in particular, it might give us the key to understanding why broad regions around criticality are observed in fMRI experiments of the brain resting state [22] . As we have shown, the system’s response is extremely large (and diverges upon increasing the network size) in a broad region of parameter space. This strongly facilitates the task of mechanisms selecting for the alleged virtues of scale-invariance and strongly suggests that a new paradigm is needed: a theory of self-organization/evolution/adaptation to the broad region separating order from chaos. In particular, GPs combined with standard mechanisms for self-organization [49] , [50] , [51] are expected to account for the empirically found dispersion around criticality [22] . This also invites the question of whether intrinsically disordered HMNs do indeed generically optimize transmission and storage of information, improve computational capabilities [19] or significantly enhance large network stability [17] , without the need to invoke precise criticality. Usually, brain networks are claimed to be small worlds; instead we have shown that large-world architectures are essential for GPs to emerge. A solution to this conundrum was provided by Gallos et al. [37] , who found that (functional) brain networks consist of a myriad of densely connected local moduli, which altogether form a large world structure and, therefore, are far from being small-world; however, incorporating weak ties into the network converts it into a small-world preserving an underlying backbone of well-defined moduli. To this end, it is essential that networks have a finite Hausdorff or fractal dimension (see Fig. 1 and Gallos et al . [37] ), confirming that finite dimensionality is a crucial feature. In this way, cortical networks achieve an optimal balance between local specialized processing and global integration through their hierarchical organization. On the other hand, weak links are not expected to significantly affect the existence of GPs. Therefore, from this perspective, (i) achieving such an optimal balance and (ii) operating with critical-like properties can be seen as the two sides of the same coin. This stresses the need to develop new models for the co-evolution of structure and function in neural networks. It is noteworthy that a mechanism for robust working memory without synaptic plasticity has been put forward very recently [52] . It heavily relies on the existence of heterogeneous local clusters of densely inter-connected neurons, where activity (memories) reverberates. Not surprisingly, this leads to power-law distributed fade-away times, which have been claimed to be the correlate of power-law forgetting [53] . This is an eloquent illustration of GPs at work. Given that disorder is an intrinsic and unavoidable feature of neural systems and that neural-network architectures are hierarchical, GPs are expected to have a relevant role in many dynamical aspects and, hence, they should become a relevant concept in Neuroscience as well as in other fields such as systems biology, where HMNs have a key role [54] . We hope that our work contributes to this purpose, fostering further research. Synthetic hierarchical networks HMN-1: At each hierarchical level l =1,2,… s , pairs of blocks are selected, each block of size 2 i −1 M 0 . All possible 4 i −1 M 0 2 undirected eventual connections between the two blocks are evaluated, and established with probability α p l , avoiding repetitions. With our choice of parameters, we stay away from regions of the parameter space for which the average number of connections between blocks n l is less than one, as this would lead inevitably to disconnected networks (as rare-region effects would be a trivial consequence of disconnectedness, we work exclusively on connected networks, that is, networks with no isolated components). As links are established stochastically, there is always a chance that, after spanning all possible connections between two blocks, no link is actually assigned. In such a case, the process is repeated until, at the end of it, at least one link is established. This procedure enforces the connectedness of the network and its hierarchical structure, introducing a cutoff for the minimum number of block-block connections at 1. Observe also that for M 0 =2 and p =1/4, α is the target average number of block-block connections and 1+α the target average degree. However, by applying the above procedure to enforce connectedness, both the number of connections and the degree are eventually slightly larger than these expected, unconstrained, values. For the HMN-2, the number of connections between blocks at every level is a priori set to a constant value α . Undirected connections are assigned choosing random pairs of nodes from the two blocks under examination, avoiding repetitions. Choosing α ≥1 ensures that the network is hierarchical and connected. This method is also stochastic in assigning connections, although the number of them (as well as the degree of the network) is fixed deterministically. In both cases, the resulting networks exhibit a degree distribution characterized by a fast exponential tail, as shown in Supplementary Fig. S1 . Empirical brain networks Data of the adjacency matrix of C. elegans are publicly available (see for example, Kaiser [32] ). Different analyses have confirmed that this network has a hierarchical-modular structure (see for example refs 33 , 39 , 40 , 55 , 56 ). In particular, in (ref. 56 ) a new measure is defined to quantify the degree of hierarchy in complex networks. The C. elegans neural networks is found to be six times more hierarchical than the average of similar randomized networks. Connectivity data for the human connectome network have been recently obtained experimentally [29] , [30] . In this case too, the network is hierarchical [22] , [33] , [42] . Supplementary Figure S2 shows a graphical representation of its adjacency matrix, highlighting its hierarchical organization. Dynamical models In both cases (Model A and Model B), neurons are identified with nodes of the network and are endowed with a binary state-variable σ=0.1. The state of the system is sequentially updated as follows. A list of active sites is kept. Model A: At each step, an active node is selected and becomes inactive σ =0 with probability μ /( λ + μ ), while with complementary probability λ /( λ + μ ), it activates one randomly chosen nearest neighbour provided it was inactive. Model B: At each step, an active node is selected and becomes inactive σ =0 with probability μ /( λ + μ ), while with complementary probability λ /( λ + μ ), it checks all of its nearest neighbours, activating each of them with probability 0<λ<1 provided it was inactive, then it deactivates. Both Model A and B have well-known counterparts in computational epidemiology, where they correspond to the contact process and the susceptible-infective-susceptible model respectively (see for instance [57] ). The value of similar minimalistic dynamic rules in Neuroscience was proven before, for example, in (ref. 58 ). Results for real networks are obtained by running Model B dynamics on the unweighted version of the network. We have verified that the introduction of weights does not alter the qualitative picture obtained. Dynamical protocols We employ four different dynamical protocols: ( i ) decay of a homogeneous state: all nodes are initially active and the system is let evolve, monitoring the density of active sites ρ ( t ) as a function of time. ( ii ) Spreading from a localized initial seed: an individual node is activated in an otherwise quiescent network. It produces an avalanche of activity, lasting until the system eventually falls back to the quiescent state; the survival probability P s ( t ) is measured. The avalanche size S is defined as the number of activation events that occur for the duration of the avalanche itself. The process is iterated and the avalanche size distribution P ( S ) is monitored. (iii) Identical to (ii), except that the seed is kept active throughout the simulation (continuous stimulus). (iv) Identical to (ii), except that the seed node is subsequently reactivated with probability p stimulus =1–exp(− r Δ t ) for t >0 (Poissonian stimulus of rate r ). Measures of response The standard method to estimate responses consisting in measuring the variance of activity in the steady-state would not provide a measure of susceptibility in the Griffiths region, where a steady-state is trivial (quiescent). We define the dynamic susceptibility as Σ( λ )= N [ ρ f ( λ )– ρ s ( λ )], where ρ f ( λ ) is the steady-state reached when a single node is constrained to be active throughout the simulation and ρ s ( λ ) the steady-state for protocol (i), that is, in the absence of constraints. In the inactive state, ρ s ( λ )=0 while ρ f ( λ ) is finite but small (of the order of 1/ N ) as the active node continuously fosters activity in its surroundings. In the active state, ρ s ( λ ) and ρ f ( λ ) are both large and again differ by a little amount (given by the fixed node and its induced activity) that vanishes for larger system sizes. Only in the parameter region where the response of the system is high, the little perturbation introduced by the constrained node produces a diverging response. This is found to occur throughout the Griffiths region (see Fig. 3 , main text), confirming the claim of an anomalous response over an extended range of the parameter λ . An alternative measure of response is provided by the dynamic range Δ, introduced by Kinouchi and Copelli [21] . We determine Δ( λ ) for various values of λ in the Griffiths and active phases, as follows: (i) a seed node is chosen and initially activated, but not constrained to be active; (ii) the dynamical model (A, B, …) is run; (iii) if the dynamics selects the seed node, and it is found inactive, it is reactivated with probability p stimulus ; (iv) the steady-state density ρ is recorded (due to the intermittent reactivation, a steady-state depending on p stimulus is always reached, unless p stimulus is infinitesimal); (v) upon varying p stimulus , the steady-state density ρ varies continuously within a finite window. We identify the values ρ 0.1 and ρ 0.9 , corresponding to the 10 and 90% values within such window, and call p 0.1 and p 0.9 the values of p stimulus leading to those values respectively; and (vi) the dynamic range is calculated as Δ=10log 10 ( p 0.9 / p 0.1 ). Notice that in the active phase ρ 0.1 reaches a finite steady-state at exponentially large times in the limit λ → λ + c . This makes the study of large systems very lengthy in that parameter region. Extended regions of enhanced response are found also by running our simple dynamic protocols on the connectome network. A way to visualize the broadening of the critical region is presented in Supplementary Fig. S3 , where the density of active sites given a fixed active seed ρ f is plotted as a function of λ . The critical region broadens if compared with the case of a regular (disorder-free) lattice of the same size. Finite-size scaling In the standard critical point scenario—assuming the system sits exactly at the critical point but it runs upon a finite system (of linear size L)—the average density (order parameter) starting from an initially active configurations decays as t −θ × exp(− t /τ( L )), where the cutoff time scales with system size, as τ( L ) n ∝ L z ( z the dynamic critical exponent), allowing us to perform collapse plots for different system sizes. Instead, in GPs, the cutoff time does not have an algebraic dependence on L ; it is the largest cluster, which is cutoff by L d , and the corresponding escape/decay time from it grows like τ( L ) ∝ exp( cL d ). Therefore, even for relatively small system sizes, such a cutoff is not observable in (reasonable) computer simulations: order-parameter-decay plots should exhibit power-law asymptotes without any apparent cutoff. On the other hand, the power-law exponent—which can be estimated from a saddle-point approximation, dominated by the largest rare region—is severely affected by finite size effects. Therefore, summing up, although in standard critical points finite size effects maintain the critical exponent but visibly affect the exponential cutoffs, in GPs, apparent critical exponents are affected by finite-size corrections while exponential cutoffs are not observable. Unless otherwise specified, simulations on HMNs are for systems of size N =2 14 =16,384. Supplementary Fig. S4 shows that upon increasing the system size (and the number of hierarchical levels accordingly), the picture of generic power-law decay of activity remains valid in the whole GP. One can observe that for each value of λ , the effective exponent tends to an asymptotic value, which is expected to hold in the large-network-size limit. Avalanches in the human connectome Unlike avalanches on synthetic HMNs, typically run on several (10 7 –10 8 ) network realizations, avalanche statistics on the human connectome network is the result of a large number of avalanches (>10 9 ) on the unique network available. Such limitation explains the emergence of strong cutoffs in the avalanche-size distributions (see Fig. 4 ). In the main text, we propose to fit avalanche size distributions with truncated power-laws, reflecting the superposition of generic power-law behaviour and finite-size effects. In order to assess the validity of our hypothesis, we resort to the Kolmogorov–-Smirnov method, by which the best fit is provided by the fitting function g ( S ), which minimizes the estimator where G ( S ) is the cumulative distribution associated with g ( S ) and F ( S ) is the cumulative distribution of empirical data (simulation results, in our case). In case of limited amount of empirical data, the use of diverse fitting techniques (least squares, maximum likelihood and so on) is advised, in order to avoid biases. However, given the abundance of data in our case, a non-linear least-squares fit provides a reliable estimate of parameters (note that a truncated power-law cannot be fit linearly by standards methods). We recall that the least-squares method is essentially a minimization problem: given a set of empirical data points ( x i , y i ) i =1,… n and a fitting function g ( x,y,b ) depending on a set of parameters b , the fit is provided by the set of parameters that minimizes the function . In the case of a linear regression, such minimization can be performed exactly. In the case of a non-linear fit, instead, the minimization has to be performed numerically. For every value of λ (every curve in Fig. 4 ), we proceed as follows: (i) we provide a least-squares fit for the avalanche-size distribution, based upon the truncated power-law hypothesis and calculate the corresponding Kolmogorov–Smirnov D KS ; (ii) we repeat the above procedure for alternative candidate distributions (non-truncated power law and exponential); (iii) we compare the results for the D KS indicators and choose the hypothesis with the smallest D KS as the best fit. In Supplementary Fig. S5 we provide an example of this procedure, as obtained from our data for λ =0.017. In this case, as in every other case examined, the truncated power law provides the best fit among the ones tested, both by the KS criterion and upon visual inspection. Notice that also the power-law hypothesis appears plausible to some extent, whereas the exponential hypothesis deviates significantly from the data; however, one chooses the minimum avalanche size S min to fit. Special attention has been devoted to the choice of the lower bound S min , as advised in (ref. 59 ). Such a choice is usually made by visual inspection for large systems, where it is easy to estimate visually the point in which power-law behaviour takes over. In small systems, instead, a more quantitative procedure is required. For every fit described above (points (i) and (ii)), we have chosen the best estimate for the S min upon preliminarily applying a KS procedure to different candidate values of S (following [59] ). We found that in each case, the KS estimator displayed a minimum for values of S ≈6, for the truncated power-law and power law hypotheses. Spectral analysis Let us call q i ( t ) the probability that the node i is active at time t . The density of active sites can be written as ρ ( t )=‹ q i ( t )›, averaged over the whole network. In the case of Model B dynamics, the probabilities q i ( t ) obey the evolution equation where A denotes the adjacency matrix and λ the spreading rate. Calling Λ a generic eigenvalue of A , its corresponding eigenvector f( Λ ) obeys A f( Λ )= Λ f( Λ ). Working on undirected networks, all eigenvalues Λ are real and any state of the system can be decomposed as a linear combination of eigenvectors, as in More importantly, if the network is connected (all our HMNs are), the maximum eigenvalue of A , Λ max , is positive and unique (Perron–Frobenius theorem, see for example, Gantmacher [60] ). As a consequence, it is commonly assumed that the critical dynamics of Equation (4) at λ = λ c is dominated by the leading eigenvalue Λ max and that, at the threshold λ c , Then one can impose the steady-state condition i ( t )=0 and, under the fundamental assumption of equation (6), derive the well-known result [44] This result relies on the implicit assumption that the principal eigenvalue is significantly larger than the following one. The existence of such spectral gap’, separating Λ max from the continuum spectrum of A , is a quite common feature in complex networks, being a measure of their small-world property. However, the picture of cortical networks as hierarchical structures distributed across several levels suggests that such systems may exhibit very different properties. We will prove this in the following and show how the above picture changes in HMNs. Figure 5a shows the average eigenvalue spectrum of the adjacency matrix A for HMNs. A detailed analysis of the peak structure is beyond the scope of this work. Notice the absence of isolated eigenvalues at the higher spectral edge (see also Fig. 5b ). The principal eigenvalue Λ max is not clearly separated from the others. The spectral gap, characterizing small-world networks, here is replaced by an exponential tail of eigenvalues. All such eigenvalues share a common feature: their corresponding eigenvectors are localized, as shown in Fig. 5c . All components are close to zero, except for a few of them in each network, corresponding to a rare region of adjacent nodes. We claim that such rare region are responsible for the emergence of the GP over a finite range of the spreading rate λ . Localization in networks can be measured through the inverse participation ratio, defined as If eigenvectors are correctly normalized, IPR ( Λ ) is a finite constant of the order of O (1) if Λ is localized, while otherwise. Such localization estimator is usually calculated for the principal eigenvalue Λ max of a network. Indeed Fig. 5d shows that IPR is finite and insensitive to changes in systems sizes. On the other hand, upon increasing the density of inter-module connections, IPR rapidly decreases, suggesting that small-world effects enhance delocalization. Having introduced a criterion to identify localized eigenvectors, we found that a whole range of eigenvalues below Λ max correspond to localized eigenvectors. The structure of equation (4) and its solutions suggest that although a spreading rate of the order of λ =1/ Λ max allows the system to access the localized behaviour dictated by the eigenvector f ( Λ max ), lager values of λ grant access to the next eigenvalues and eigenvectors that are less and less localized. This ultimately establishes a strong connection between eigenvalue localization and rare-region effects. How to cite this article: Moretti, P. and Muñoz, M. A. Griffiths phases and the stretching of criticality in brain networks. Nat. Commun. 4:2521 doi: 10.1038/ncomms3521 (2013).